Liquid–liquid transition in a strong bulk metallic glass-forming liquid Polymorphic phase transitions are common in crystalline solids. Recent studies suggest that phase transitions may also exist between two liquid forms with different entropy and structure. Such a liquid–liquid transition has been investigated in various substances including water, Al 2 O 3 -Y 2 O 3 and network glass formers. However, the nature of liquid–liquid transition is debated due to experimental difficulties in avoiding crystallization and/or measuring at high temperatures/pressures. Here we report the thermodynamic and structural evidence of a temperature-induced weak first-order liquid–liquid transition in a bulk metallic glass-forming system Zr 41.2 Ti 13.8 Cu 12.5 Ni 10 Be 22.5 characterized by non- (or weak) directional bonds. Our experimental results suggest that the local structural changes during the transition induce the drastic viscosity changes without a detectable density anomaly. These changes are correlated with a heat capacity maximum in the liquid. Our findings support the hypothesis that the ‘strong’ kinetics (low fragility) of a liquid may arise from an underlying lambda transition above its glass transition. There is a growing interest in density- or entropy-driven liquid–liquid phase transitions (LLTs) [1] , [2] , [3] , [4] , [5] . The LLT of two distinct forms of liquid water has been intensely studied and debated [1] , [2] , [3] , [4] , [5] , [6] , [7] . Not limited to water, experimental and numerical support for existence of a polyamorphism or LLT has also been found in other systems, for example, in triphenyl phosphate [1] , [2] , Y 2 O 3 -Al 2 O 3 (refs 3 , 4 ), Si [5] , SiO 2 (refs 6 , 7 ), BeF 2 (ref. 8 ), Ge [9] and Ce-Al [10] , [11] . Most of the LLTs occur in the supercooled liquid state. In the case of the molten phosphorus (P), the LLT takes place far above its melting point in the stable liquid state [12] . Even though there is growing evidence for the existence of a LLT, the nature of the transition still remains ambiguous, as it is either hidden by crystallization or located at high temperature and high (or even negative) pressure, which is challenging for experimental observation. To this end, computer simulations are usually employed to investigate the elusive LLT. In a parallel approach, the lambda (order–disorder) transition phenomena [13] have been studied and compared with the liquid–liquid critical point (LLCP) simulations using Jagla model [14] . It was found that a LLT on a LLCP is reminiscent of a lambda transition characterized by a divergence in the correlation length with a λ-shape heat capacity peak. LLCP is a pressure–temperature combination where the difference between two phases disappears and the phase transition becomes continuous as crossing the point. In an experiment or simulation, measurements were usually carried out in the first-order transition region crossing a phase boundary or in the supercritical region where the lambda transition was smeared out. The underlying LLCP is often located by an extrapolation of the equilibrium phase boundary, known as the coexistence line or tracing back the response function (for example, heat capacity) maximum, the Widom line. One important approach to exploring a LLT is to study the heat capacity behaviour that characterizes the entropy fluctuation of the system. The heat capacity of supercooled water exhibits a large and increasing value at ~240 K and a small value at ~150 K, between which experimental data are not available due to crystallization [15] . Simulations and experiments [16] , [17] of nanoconfined water suggest a lambda-like heat capacity peak between the two temperatures that separates a high-density liquid near the melting temperature T m from a low-density liquid near its T g . In analogy to water, heat capacity maxima have been also found at high temperature far above the melting point in simulations of the network glass-forming liquids SiO 2 (refs 6 , 7 , 18 ) and BeF 2 (refs 8 , 18 ). More interestingly, the suggested transitions in these systems are found to relate to an anomalous change in dynamic properties of liquids, known as a strong-fragile crossover or transition [7] , [8] , [15] , [19] , [20] . This refers to a drastic change in the temperature dependence of relaxation processes (for example, viscosity) between an Arrhenius-like (strong) and a non-Arrhenius (fragile) behaviour. The magnitude of the deviation from the Arrhenius law can be described by the terms ‘strong’ and ‘fragile’ in the classification scheme of the ‘fragility’ concept proposed by Angell [21] , but the origin of fragility has been a long-standing puzzle. The understanding of the strong-fragile crossover may decipher the origin of the liquid fragility that is of great fundamental and practical importance to glasses and liquids. Recently, a hypothesis has been proposed that the strong liquids differ from fragile liquids by occupying opposite flanks of an underlying lambda transition [13] . It has an important implication that strong liquids are such systems where a LLT can be observed above (not below) its glass-transition temperature, T g , at appropriate pressure [13] , as implied in the studies of water, SiO 2 and BeF 2 . In contrast to the network glass formers, metallic glass formers are characterized by the non-(or weak) directional bonds in the melt [22] . However, there is direct and indirect evidence of the existence of a strong-fragile crossover [23] , [24] in bulk metallic glass (BMG)-forming liquids. This makes them of great interest to be studied to test the hypothesis of underlying lambda transitions that was originally based on simulations and network glass formers. We choose the BMG-forming system, Zr 41.2 Ti 13.8 Cu 12.5 Ni 10 Be 22.5 (Vit.1) as a model system for experimental investigations of a possible LLT, because it is an archetypal strong BMG system and exhibits a change in the viscosity of approximately two orders of magnitude in the equilibrium melt, which has been attributed to a reversible, temperature-induced strong-fragile crossover [23] . In the Vit.1 system, the strong-fragile crossover upon heating takes place above the melting point, which provides a unique opportunity for thermodynamic studies using conventional calorimetric methods. Thus, we carry out high-temperature calorimetric experiments and observe an anomalous lambda-like heat capacity peak in the stable liquid state. Furthermore, we investigate the structural changes corresponding to the thermodynamic and dynamic anomalies with the in situ synchrotron X-ray-scattering experiments in contactless environment using an electrostatic levitator (ESL). We show thermodynamic and structural evidence that is consistent with the observations in viscosity, suggesting that there is a LLT from one liquid phase to another with different entropy, local structures and fragility in the Vit.1 system. 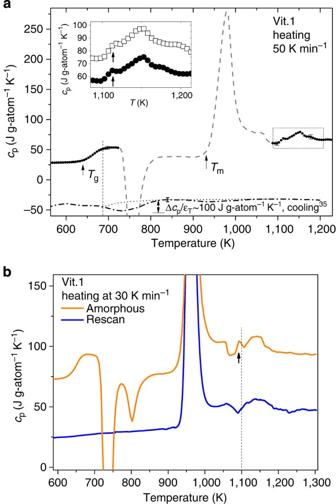Figure 1: Heat capacitycpof Vit.1. (a)cpof an amorphous sample is measured upon heating at 50 K min−1. Solid circles represent the glassy, supercooled liquid and stable liquid states; the dashed curve indicates the crystallization and melting processes. Note that there is a heat capacity peak at around 1,100–1,200 K, which occurs in the molten liquid according to thein situXRD taken at a 10 times higher heating rate (~9 K s−1) (seeFig. 2). Inset shows the magnification of thecppeak (1,100–1,200 K) where the solid circles and open squares represent two separate measurements (vertically shifted for clarity). The arrows indicate that there is a small subpeak on the left shoulder of the main peak. In the lower part of the figure, the dash-dot curve shows the heat capacity during cooling of Vit.1 taken fromcp/εTin Ohsakaet al.35(assuming the emissivity35εT=0.18), which is here plotted as negative values to indicate the exothermic event around 700–800 K in the supercooled liquid region in reference to the baseline (dotted curve) (see Discussion). (b)cpmeasured upon heating at 30 K min−1for the amorphous sample (upper) and once-melted crystallized sample (lower) (vertically shifted for clarity). The arrow shows the small subpeak separated from the main peak to a lower temperature. Heat capacity maximum Figure 1 shows the heat capacity ( c p ) of Vit.1. A heat capacity peak is observed on heating between around 1,100 and 1,200 K, above the reported [25] liquidus temperature 1,026 K. The area of the c p peak is proportional to the heat gain, which is determined to be Δ H LL ≈1.0±0.1 kJ g-atom −1 , about 10% of the enthalpy of fusion (Δ H f ≈9.7±0.7 kJ g-atom −1 ). The inset shows the zoom-in of the peak (solid circles) and a separate scan (open squares) in which the main peak is reproduced (1,100–1,200 K). We notice that a small subpeak on the left shoulder of the broad peak is also reproducible. By lowering the heating rate down to 30 K min −1 , this small subpeak can be separated to a lower temperature <1,100 K from the main broad peak (see the upper curve in Fig. 1b ). And during a rescan of the once-melted crystallized sample, the subpeak disappears while the main peak remains (lower curve in Fig. 1b ). This observation suggests that this small subpeak probably comes from a small portion of remaining crystalline phases. The first scan apparently reduces the inhomogeneity and thus diminishes the small subpeak and ruggedness of the measured heat capacity curve. However, we show in the next section that the broad main peak cannot be explained by melting of crystals and should be considered as a consequence of an intrinsic change in the liquid. Figure 1: Heat capacity c p of Vit.1. ( a ) c p of an amorphous sample is measured upon heating at 50 K min −1 . Solid circles represent the glassy, supercooled liquid and stable liquid states; the dashed curve indicates the crystallization and melting processes. Note that there is a heat capacity peak at around 1,100–1,200 K, which occurs in the molten liquid according to the in situ XRD taken at a 10 times higher heating rate (~9 K s −1 ) (see Fig. 2 ). Inset shows the magnification of the c p peak (1,100–1,200 K) where the solid circles and open squares represent two separate measurements (vertically shifted for clarity). The arrows indicate that there is a small subpeak on the left shoulder of the main peak. In the lower part of the figure, the dash-dot curve shows the heat capacity during cooling of Vit.1 taken from c p / ε T in Ohsaka et al. [35] (assuming the emissivity [35] ε T =0.18), which is here plotted as negative values to indicate the exothermic event around 700–800 K in the supercooled liquid region in reference to the baseline (dotted curve) (see Discussion). ( b ) c p measured upon heating at 30 K min −1 for the amorphous sample (upper) and once-melted crystallized sample (lower) (vertically shifted for clarity). The arrow shows the small subpeak separated from the main peak to a lower temperature. Full size image Monitoring melting by in situ X-ray diffraction Although the liquidus temperature was determined [25] to be 1,026 K using calorimetry, it needs to be investigated here whether the c p peak (1,100–1,200 K) upon heating occurs in the stable liquid state or is due to melting of some remaining crystalline phases. We performed in situ X-ray diffraction (XRD) experiment on levitated Vit.1 droplets (see Methods). The XRD patterns of Vit.1 recorded on continuous heating at a rate of about 9 K s −1 are shown in Fig. 2 . It is seen that the sharp Bragg peaks first appear due to the crystallization of the amorphous sample and then disappear by melting. As the temperature increases up to around 1,091 K, the sharp peaks disappear in both the 1st and 2nd maxima of diffraction curves, indicating that the crystals were molten. This corresponds to the pronounced endothermic peak observed at 939–1,080 K on the c p curve in Fig. 1 . It is possible that there still remains a tiny portion of crystalline particles that melt above 1,100 K. However, for the broad c p peak in the temperature range ~1,100–1,200 K, if it was due to melting of remaining crystals, the crystalline volume fraction would be around 10% of the liquid according to the ratio of the enthalpy change by this c p peak to the heat of fusion (Δ H LL /Δ H f ≈10%). This amount of crystals would be well within the detection limit and should be clearly seen as pronounced sharp Bragg peaks in XRD patterns over the entire range of the c p peak. In contrast, according to the integral diffraction patterns between 1,091 and 1,200 K in Fig. 2 , it is unlikely that there (1,100–1,200 K) still remained 10% crystals of the system. If the crystals would be very small, such as nano-crystalline particles, there is a possibility that only broad maxima rather than sharp Bragg peaks appear in the diffraction patterns. However, our volume measurements show no indication of the presence of a nano-crystalline or crystalline phase (see Discussion). 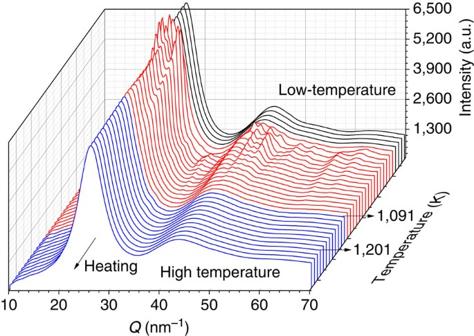Figure 2:In situsynchrotron XRD integral patterns of Vit.1 upon heating. As the temperature increases, the amorphous sample is crystallized and the Bragg peaks become pronounced. When the melting sets in, these sharp peaks decline and disappear. The blue colour highlights the patterns corresponding to the temperature range where thecppeak is observed (1,100–1,200 K). Figure 2: In situ synchrotron XRD integral patterns of Vit.1 upon heating. As the temperature increases, the amorphous sample is crystallized and the Bragg peaks become pronounced. When the melting sets in, these sharp peaks decline and disappear. The blue colour highlights the patterns corresponding to the temperature range where the c p peak is observed (1,100–1,200 K). Full size image The heat capacity c p peak is observed in nearly the same temperature range (1,100–1,200 K) where the viscosity drops anomalously by approximately two orders of magnitude [23] . During the drastic viscosity change, there is a large change in the temperature dependence of viscosity, which can be described by the Vogel–Fulcher–Tammann equation η = η 0 exp[ D * T 0 /( T – T 0 )], where η is viscosity and η 0 is constant [26] . The fitting parameter D* characterizes the fragility of the liquid, which changes significantly from D *=26.5 below 1,100 K to D *=12 above 1,200 K in the present liquid [23] . This indicates a crossover of dynamics from the strong to fragile liquid (see Fig. 8 of Way et al. [23] ). It appears that the heat capacity peak is associated with this crossover of liquid dynamics, which, by a semi-quantitative estimation, also leaves out the alternative explanations of the viscosity hysteresis based on crystalline particles. If we assume that there were remaining about 10% crystals melted throughout the c p peak, the crystalline particles in the liquid can be modelled as concentrated suspensions of solid spheres. According to the models [27] , [28] for the viscosity behaviour of suspensions of solid spheres based on extensive experimental data, for the melting of 10% crystals, the viscosity change of the entire system would be around 150% (see Fig. 1 of Thomas [27] and Fig. 4 of Frankel and Acrivos [28] ), which cannot explain the measured change in viscosity of approximately two orders of magnitude, that is, 10,000% in the present system. 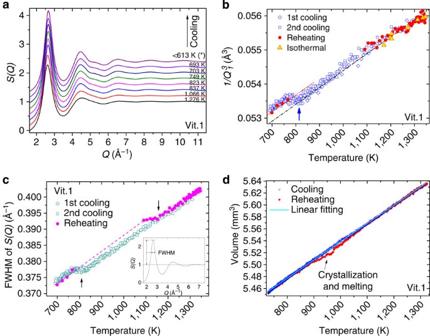Figure 3: Structural changes in the liquid and volume measurements. (a) Examples of total structure factorS(Q)on cooling from about 1,300 K to ~610 K. (*) marks the glassy state. The structure factors are vertically shifted for clarity. SeeSupplementary Fig. S1for more structure factors. (b) Temperature dependence of1/Q13(Å3) on cooling (blue diamonds and squares) and heating (red dots). Filled yellow triangles are isothermal measurements on stepwise heating. The arrow points out a clear discontinuity of1/Q13upon cooling at around 830 K. The lower and upper lines are the data fittings with Yavari’s equation (see text) for two liquid states. (c) The FWHM of the 1st peak ofS(Q)(see inset) versus temperature during thermal cycles. The arrows point out the clear slope changes in the temperature range 760–830 K during cooling and 1,100–1,200 K upon reheating. The dashed line is the assumed heating data trace if crystallization can be avoided on reheating. (d) Macroscopic liquid volume measured in the ESL during cooling and reheating. The deviation of the macroscopic volume (density) data on reheating (arrow) from the data on cooling is due to the process of partial crystallization and re-melting at around 800–1,100 K, which is the temperature range where the XRD data for the liquid state are not available on reheating, seen as a data gap between the solid circles inbandc. Figure 3: Structural changes in the liquid and volume measurements. ( a ) Examples of total structure factor S(Q) on cooling from about 1,300 K to ~610 K. (*) marks the glassy state. The structure factors are vertically shifted for clarity. See Supplementary Fig. S1 for more structure factors. ( b ) Temperature dependence of 1/Q 1 3 (Å 3 ) on cooling (blue diamonds and squares) and heating (red dots). Filled yellow triangles are isothermal measurements on stepwise heating. The arrow points out a clear discontinuity of 1/Q 1 3 upon cooling at around 830 K. The lower and upper lines are the data fittings with Yavari’s equation (see text) for two liquid states. ( c ) The FWHM of the 1st peak of S(Q) (see inset) versus temperature during thermal cycles. The arrows point out the clear slope changes in the temperature range 760–830 K during cooling and 1,100–1,200 K upon reheating. The dashed line is the assumed heating data trace if crystallization can be avoided on reheating. ( d ) Macroscopic liquid volume measured in the ESL during cooling and reheating. The deviation of the macroscopic volume (density) data on reheating (arrow) from the data on cooling is due to the process of partial crystallization and re-melting at around 800–1,100 K, which is the temperature range where the XRD data for the liquid state are not available on reheating, seen as a data gap between the solid circles in b and c . 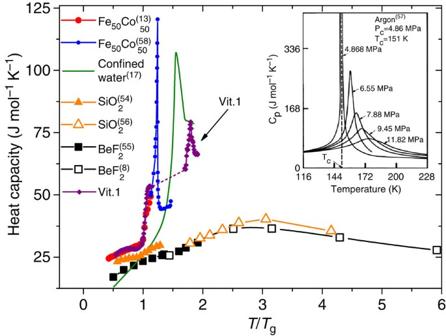Figure 4: Comparison of heat capacity maxima between the liquid Vit.1 and other glass formers. Solid and open symbols represent experimental and simulation data, respectively (the last data point of SiO2is extracted13from Fig. 3 of Scheidleret al.52). The heat capacity values are plotted against theTg-scaled temperature. For both SiO2and BeF2, the heat capacity maxima with the dynamic crossover are located beyond the normal measurement range, far aboveTm, suggesting that the liquid–liquid transitions are in the stable liquid state at the high temperature. In the case of water, the suggested liquid–liquid transition is in the supercooled liquid regime where thecppeak is observed in the water confined by nanopores to avoid crystallization. The liquid–liquid transition of Vit.1 upon heating is aboveTmand has a sharpercppeak than that of SiO2and BeF2. These liquid–liquid transitions are considered as off-critical phenomena, comparing with the critical phenomenon of the lambda transition in the non-liquid superlattice Fe50Co50with a very sharp lambdacppeak. Inset: the heat capacity of argon13,54appears in various forms around its liquid–gas critical point at different pressures. (Parts of the figure are reproduced from Weiet al.13). Full size image Figure 4: Comparison of heat capacity maxima between the liquid Vit.1 and other glass formers. Solid and open symbols represent experimental and simulation data, respectively (the last data point of SiO 2 is extracted [13] from Fig. 3 of Scheidler et al. [52] ). The heat capacity values are plotted against the T g -scaled temperature. For both SiO 2 and BeF 2 , the heat capacity maxima with the dynamic crossover are located beyond the normal measurement range, far above T m , suggesting that the liquid–liquid transitions are in the stable liquid state at the high temperature. In the case of water, the suggested liquid–liquid transition is in the supercooled liquid regime where the c p peak is observed in the water confined by nanopores to avoid crystallization. The liquid–liquid transition of Vit.1 upon heating is above T m and has a sharper c p peak than that of SiO 2 and BeF 2 . These liquid–liquid transitions are considered as off-critical phenomena, comparing with the critical phenomenon of the lambda transition in the non-liquid superlattice Fe 50 Co 50 with a very sharp lambda c p peak. Inset: the heat capacity of argon [13] , [54] appears in various forms around its liquid–gas critical point at different pressures. (Parts of the figure are reproduced from Wei et al. [13] ). Full size image Structural changes on cooling and reheating Besides monitoring the melting in the vicinity of liquidus temperature, in situ synchrotron XRD combined with ESL is able to study the structural changes with temperature cycles (700–1,300 K) during continuous cooling and reheating of the sample, as well as at different constant temperatures. One particular advantage of ESL is the ability to access the deeply supercooled regime due to the absence of heterogeneous nucleation sites, for example, container walls. Thus, it allows us to explore a possible structural transition in the supercooled state, which is usually hidden by crystallization and difficult to detect with conventional methods. Electrostatically levitated droplets were cooled from >1,300 K down to <700 K. The XRD patterns were recorded and the total structure factor S(Q) was extracted from the diffracted intensity data (see Methods). A few examples of S(Q) on cooling are shown in Fig. 3a . The first peak position of the structure factor, Q 1 , corresponds to the length scale of medium-range order correlations in real space [29] . In Fig. 3b , the 3rd power of the inverse of Q 1 ( 1/Q 1 3 in the volume dimension (Å 3 )) on cooling is plotted as open symbols (diamonds and squares) against temperature. As expected, 1/Q 1 3 shifts to smaller values with decreasing temperature. However, it is clearly observed that a sudden change in the temperature dependence of 1/Q 1 3 occurs around 830 K (arrow in Fig. 3b ). During undercooling, the data (open diamonds and squares) deviates from its original high- Q 1 state (lower line) and shifts discontinuously (see arrow) to a low- Q 1 state (upper line) between around 830 and 760 K. With further decreasing temperature, the data retain their low- Q 1 state. For Vit.1, there are 15 different pairs of partial structure factors that contribute to the measured total structure factor S(Q) , weighted by their corresponding X-ray-scattering cross-sections. However, Zr has the highest concentration in Vit.1 and the largest atomic number. Therefore, the Zr-X (X=Zr, Cu, Ti, Ni) spatial correlations dominate the contribution to the first peak of S(Q) . The discontinuity in 1/Q 1 3 observed in Fig. 3b suggests an abrupt change in the Zr-dominant interatomic correlations in real space. Note that T g of Vit.1 is located at a much lower temperature [30] (<700 K). Therefore, the discontinuity observed at around 830 K cannot be attributed to the approaching of the glass transition. The X-ray diffractogram is recorded further upon reheating of the sample. The solid circle symbols from 700 to 770 K and from 1,091 to 1,350 K in Fig. 3b represent 1/Q 1 3 on reheating. The values of 1/Q 1 3 upon reheating reproduce the values during cooling for each respective temperature range, except for the range from 770 to 1,091 K. In this temperature interval (770–1,091 K), the sample devitrified and measurements on the liquid state are not possible. The crystallization upon reheating beginning at 770 K is expected if the (re-)heating rate of the supercooled liquid is not so fast as to avoid the crystallization altogether (<200 K s −1 ), according to the time-temperature-transformation diagram of Schroers et al. [31] . It should be pointed out that a discontinuity in 1/Q 1 3 upon reheating is not obvious in the temperature range, where the c p peak is observed around 1,100–1,200 K, from the limited data points collected, due to the narrow time window of the detection. Nevertheless, it appears that once the sample is molten at ~1,100 K, it recovers its high- Q 1 state (lower line), distinct from its low- Q 1 state (upper line). Figure 3c shows the full width at half maximum (FWHM) of the first peak of S(Q) as a function of temperature during cooling and reheating cycles. It is clearly observed that an abrupt change of the FWHM during cooling (open symbols) has occurred around 760–830 K, below which the data shift to a distinct upper track while return to the decreasing trend. This is the exactly same feature as the sudden change observed in 1/Q 3 in Fig. 3b . Furthermore, on reheating, the data points (solid symbols) traced back the cooling data in the temperature range of ~700–770 K. As expected, a data gap is left due to interference of crystallization and re-melting on reheating. After the system returns to the liquid state at high temperature (~1,100 K), the data points exhibit a clear change of slope at around ~1,150 K, which corresponds to the temperature range where the c p peak is observed in the calorimeter ( Fig. 1 ). It is striking that the changes on cooling and reheating appear as a reversible phenomenon, and the data in Fig. 3c display a form of three quarters of a hysteresis when the missing data gap is extrapolated as the dashed line from the lower temperature data. FWHM is a parameter for characterizing the diffraction peak shape and shows a lower degree of scatter of data points than Q 1 , because for determining Q 1 , the error may rise by the spline analysis procedure. FWHM provides more accurate characterization of structural changes and thus allows us to see the sudden change at high temperature (~1,150 K) as expected from c p and the viscosity measurements. Macroscopic liquid volume and density We further found that the transition in the atomic scale structure is not reflected in the macroscopic liquid volume (or density) measured in ESL ( Fig. 3d ). The volume data appear as a continuous function of temperature, and no anomaly is observed in the temperature range 760–830 K on cooling (blue triangles) or 1,100–1,200 K on heating (red diamond). This phenomenon can be understood by considering that liquids are distinct from amorphous solids by the fact that liquids are not rigid and the atomic structures of a liquid behave differently at different length scales. The increase of the local volume observed on one length scale can be accompanied by a decrease on another length scale, which, however, may be out of our observation window (see Supplementary Fig. S3 ). Thus, the local volume change does not necessarily result in liquid volume (density) change, which averages over a macroscopic volume (~5 mm 3 ). One must emphasize that the deviation of the volume data on heating (see arrow) is due to partial crystallization, irrelevant to the LLT, although it has been previously confused with a strong-fragile hysteresis [32] . By a linear fitting, the volume measurement reveals a constant volume thermal expansion coefficient α macro ≈5.56 × 10 −5 K −1 , which is remarkably smaller than α XRD ≈9.20 × 10 −5 K −1 on the microscopic scale obtained from the XRD measurement when applying Yavari’s equation [33] ( Q 1 ( T 0 )/ Q 1 ( T )) 3 =1+ α XRD ·( T − T 0 ) (see Methods). This discrepancy is expected for T > T g because the Yavari’s approach is based on the underlying pre-assumption that the structural change at T < T g is negligible, which is no longer valid in the cases of the liquid state ( T > T g ), as discussed in Mattern et al. [34] . In liquids, the thermal expansion coefficient is varying on different length scales. The c p peak shown in Fig. 1 is measured upon heating using a calorimeter. It should be noted that the c p measurement of deeply supercooled liquid is not possible for the calorimeter, because the crucible walls act as potent heterogeneous nucleation sites for the liquid. Thus, containerless techniques such as electrostatic levitation are necessary to access the deep supercooled region. The dash-dot line in the lower part of Fig. 1 is the deep supercooled c p data from c p / emissivity extracted from a temperature-time profile measured in an ESL by Ohsaka et al. [35] . An exothermic peak is reported around 700–800 K corresponding to an enthalpy release ~900 J g-atom −1 estimated by the authors, which, by the following analysis alternative to the authors’, should be associated with the c p peak on heating (1,100–1,200 K) when taking the viscosity hysteresis and structural measurements into account. Both c p peaks correspond to a similar enthalpy change (~1 kJ g-atom −1 ) and form a hysteresis with respect to temperature, which is comparable to the viscosity hysteresis that characterizes the strong-fragile crossover [23] . The correlation between thermodynamics and kinetics is suggested by Adam–Gibbs theory [36] , at least, qualitatively ( Supplementary Discussion ). These hysteresis are consistent with the hysteresis-like behaviour in 1/Q 1 3 and FWHM of the structure factor S(Q) ( Fig. 3b ) where two different local structures correspond to the different properties. These findings suggest that there exists a reversible LLT between two liquid phases with different entropy, liquid dynamic fragility and local structures in the investigated system. Alternative explanations to the LLT could be crystallization or chemical decomposition (phase separation) for the anomalies in the supercooled multicomponent liquid Vit.1. If we assume the sudden changes in S(Q) ( Fig.3b ) during cooling are due to crystallization, we should be able to see Bragg peaks in the XRD patterns. However, the complete XRD data set during cooling from ~1,300 K (see Fig.3a and Supplementary Fig. S1 ) show no crystalline reflexes during the entire cooling process, indicating that no crystallization has occurred. Furthermore, the Bragg diffraction peaks would keep increasing as the crystals grow. However, the sudden changes observed in S(Q) take place only in a certain temperature range 760–830 K and clearly ends at around 760 K. This is very different behaviour from crystallization. It could be supposed that the anomalies observed during cooling at ~800 K and upon heating at ~1,150 K are due to the respective formation and melting of nano-crystals, which are so small that they do not raise sharp Bragg diffraction peaks but only broad diffuse maxima in the scattering patterns. In such a case, it is not clear how the drastic viscosity change in the liquid could be caused by such a small portion of nano-crystals [27] , [28] . Moreover, according to literature values [35] , the volume change for the transformation from the liquid to the crystalline state of Vit.1 can be calculated to be 1.29% at ~800 K and 1.82% at ~1,150 K by linear extrapolation. From the rule of mixing, ρ mix = ρ liq (1− x )+ ρ cry x where ρ is density and x is (nano-) crystalline volume fraction, one can derive the equation for volume change ( V liq − V mix )/ V liq =1−1/{1+ x [( V liq − V cry )/ V cry ]}. The values of the ratio V liq / V cry = ρ cry / ρ liq can be obtained from Ohsaka et al. [35] , and the density of nano-crystals is approximated to that of crystals. Consequently, the system volume changes by 10% nano-crystalline volume fraction, estimated by the c p peaks area ratio, would be around 0.13% at 800 K and 0.19% at 1,150 K, which would correspond to the values of changes in Fig. 3d , approximately 0.007 and 0.010 mm 3 , respectively. However, no such change is observed around these temperatures ( Fig. 3d ), which is contrary to the nano-crystal or crystal scenario. Phase separation is a common phenomenon in multicomponent systems, during which the system decomposes into two (or more) immiscible phases with different compositions, which is in contrast to a LLT where one liquid phase transforms into another completely. Vit.1 has been extensively studied near T g by Loffler et al. [37] and Schneider et al. [38] , [39] using small-angle neutron scattering (SANS). They reported interference maxima in the scattering intensity, giving evidence for spinodal decomposition on the nanometre scale in the amorphous phase upon annealing near T g , which is followed by nanocrystallization. These results have been later challenged by Hono and coworkers [40] by showing that no evidence for decomposition before the crystallization of icosahedral phase was observed using transmission electron microscopy, small-angle X-ray scattering and high-resolution three dimensional atom probe. Interpretations of these results appear controversial. For the case reported by Hono and coworkers, crystallization seeded from a single amorphous phase rather than immiscible separated phases, indicating that no decomposition occurs in the supercooled liquid. For the case reported by Loffler et al. [37] and Schneider et al. [38] , [39] , we note that the intensity maximum in SANS occurred from room temperature up to a critical temperature T c ~670 K, above which no maximum was observed. In addition, the reported decomposition triggered nanocrystallization after an incubation time, which was a decreasing function with increasing temperatures (2.8 s at 661 K) according to Loffler and Johnson’s model [41] . In contrast, the sudden change in S(Q) observed in the present study, as well as the exothermic c p peak reported by Ohsaka et al. [35] , is well above the critical temperature for decomposition, and no crystallization is detected by in situ XRD. Therefore, the LLT suggested in this work is not related to the decomposition, which might occur at lower temperatures near T g as suggested in Loffler et al. [37] and Schneider et al. [38] . If we assume a scenario including a phase separation, one would expect the presence of two glass transitions corresponding to two separated phases; however, no such indication has been observed in the present calorimetric measurements or reported studies to the best of our knowledge. At last, we emphasize that the LLT is not an exclusive phenomenon of phase separation. Both phenomena can occur simultaneously when the composition of the system is not right on the critical composition for a pure polyamorphic transition. In this case, it is conceivable that the high-temperature fragile phase separates into two phases: one is strong and the other remains fragile. A slight compositional change does not affect the intrinsic liquid structural change, which is the real origin of the drastic viscosity and fragility change of the liquid. This is analogous to the first-order order–disorder transition system Cu 3 Au where the order–disorder transition and the phase separation occur simultaneously with decreasing temperature when the composition of Cu-Au is slightly off the ratio 3:1. For Vit.1, the volume data obtained by cooling from the high-temperature liquid ( Fig. 3d ) are fitted well by a linear function, yielding a constant thermal expansion coefficient, which indicates that the compositional change must be so small (if not zero) that it cannot result in a detectable change in thermal expansion coefficient. Thus, the drastic viscosity change should not be explained by a demixing but is more likely caused by intrinsic changes in short- and/or medium-range order atomic configurations of the liquid. According to the above analysis, it is plausible to consider the LLT that involves the intrinsic structural changes of the liquid itself for a reasonable explanation of the anomalies in Vit.1. The hysteresis phenomena pronounced in viscosity [24] , the heat capacity peaks ( Fig. 1 ) and the changes in structure factor S(Q) ( Fig. 3b ) suggest a weak first-order character of the LLT between the two liquids, in which the high-temperature liquid needs to be supercooled and the low-temperature liquid needs to be overheated to nucleate the respective other liquid. We propose a homogeneous nucleation scenario for the mechanism of the LLT suggested here. On heating, the fragile droplet nucleates homogeneously in the strong liquid matrix at ~1,100 K. On cooling, the reversible transition occurs at ~830 K through the homogeneous nucleation of strong liquid droplets in the fragile liquid matrix. Apparently, there is considerable undercooling and overheating involved, where a faster cooling rate may cause a lower transition temperature. Thus, the structural transition during cooling at a rate of ~10 K s −1 in ESL is detected at a somewhat lower temperature (~800 K) than the kinetic fragile-to-strong transition (~900 K) observed at a cooling rate of ~2 K s −1 in the viscosity measurements. According to the classic nucleation theory, the homogeneous nucleation rate depends on both the diffusion (viscosity) and the energy barrier for the critical nucleus, Δ G * /Δ , where γ LL Δ S LL is the fragile/strong liquid interfacial energy, Δ S LL is the entropy difference across the interfaces and Δ T c is either the critical undercooling Δ T c u or overheating Δ T c o . In this scenario, if the critical temperature T c for the first-order LLT (Δ G LL =0) is assumed to be located approximately in the middle between 830 and 1,100 K at 965 K (with Δ T c u =Δ T c o =135 K), the entropy difference between the strong and fragile liquid can be estimated as Δ S LL ≈1 J g-atom −1 K −1 . This makes it at first surprising that large undercooling (overheating) is necessary to overcome this barrier. However, it needs to be emphasized here that Vit.1 exhibits a very sluggish liquid kinetics, which results in both slow nucleation and growth kinetics of the respective other liquid phase, even with a rather small barrier for homogeneous nucleation. One fundamental difference compared with a first-order liquid-crystalline transition has to be pointed out. During melting of a crystalline solid, the liquid forms spontaneously at internal interfaces, such as grain boundaries, and at the surface by heterogeneous nucleation of the melt, and virtually no overheating is observed. In contrast, in the strong liquid that transforms into the fragile liquid, few internal interfaces exist and heterogeneous nucleation is rare, leading to overheating in this case. In the pressure–temperature ( P–T ) phase diagram, the slope of the liquid–liquid phase equilibrium line between the strong and fragile phases can be determined by the Clausius–Clapeyron relation, d P /d T =Δ S LL /Δ V LL . As shown in Fig. 3d , no abrupt density change (that is, Δ V LL ≈0 mm 3 ) is observed during the LLT. This suggests an infinite slope of tangent of the coexistence line at P =1 atm (that is, d P /d T =Δ S LL /Δ V LL ≈∞ K GPa −1 ) that separates two phases. If the P–T phase diagram of Vit.1 resembles that of water [42] , silica [43] and Al 2 O 3 -Y 2 O 3 (ref. 4 ), where the coexistence line terminates at a hypothesized LLCP with decreasing pressure (sometimes to negative values), the LLCP for Vit.1 is expected <1 atm or at a negative pressure. In contrast, the Jagla model [14] displays an opposite trend of the coexistence line that terminates at the LLCP with increasing pressure. Vit.1, if having the same characteristic as the Jagla model, would have a LLCP at higher pressures >1 atm. In an experimental detection, a first-order phase transition may not occur at the coexistence line because one phase can remain supercooled or overheated metastable state until a stability limit (spinodal) is approached. In the present case, the hysteresis in the c p peak and changes of S(Q) suggest that the spinodals for strong and fragile phases lie at temperatures ≥1,100 and ≤830 K, respectively. The enthalpy change for the LLT of Vit.1, around 1.0 kJ g-atom −1 , is about 10% of enthalpy of fusion. Comparing with LLT in Si, which has an enthalpy change [44] of 5.5 kJ g-atom −1 for the Stillinger–Weber potential (or 6 kJ g-atom −1 from ab intio calculation), both LLTs have the similar fraction of enthalpy of fusion, that is, ~10–11%. (enthalpy of fusion of silicon [45] : ~50.6 kJ g-atom −1 ). Comparing with the liquid–crystal transition, the enthalpy and entropy changes for the LLT are quite small. This leads to the fact that the energy barrier for the LLT is much smaller than that for the liquid–crystal transition. In such a case, the strong liquid phase as an intermediate state between the fragile liquid and the crystalline phase can stay stably in a considerable temperature range after the LLT rather than crystallize immediately, which is one important reason (another is kinetics) why Vit.1 can be readily deeply supercooled to the region where a strong phase can be observed without the interference of crystallization. The enthalpy difference for the LLT of Al 2 O 3 -Y 2 O 3 is about 35–55% of enthalpy of fusion [4] , suggesting that the low-temperature liquid phase is relatively vulnerable to crystallization. That is probably why crystallization is lastly not avoided during cooling even in a containerless environment [4] . The sudden change in structure factors observed around 830 K during continuous cooling in Fig. 3b can be interpreted as the transition from a smaller to a larger length scale state (high- Q 1 state→low- Q 1 state) of Zr-dominant correlations. If we assume that the number and species of atoms on the measured length scale keep constant, a transition from a smaller to larger length scale state implies the change in local atomic packing from a denser to looser state. To obtain the real space structural information, the reduced total pair distribution functions G(r) are calculated from the structural factor S(Q) by Fourier transform [46] . The n th peak position of G(r) reflects the n th coordination shell distance r n . No kink is observed around 800 K in the first three coordination shell distances from G(r) during cooling, and the data for the 4th (or n th≥4th) shell include too much noise to make any conclusion (see Supplementary Figs. S2, S3 ). Thus, the length scale of the structural transformation in the supercooled state is likely not less than the 4th shell distance (≥1 nm) and can be reflected in by Q 1 of S(Q) in reciprocal space ( Fig. 3b ), which is demonstrated to be more sensitive to medium/long range correlations [29] . It is hardly a coincidence that the length of the ideal face-centered-cubic (FCC)-like cluster-unit-cell for the medium-range order of Miracle’s efficient cluster packing model [47] is calculated to be around 1.0–1.3 nm. The FWHM of S(Q) ( Fig. 3c ) is a complementary parameter for the structural characterization to Q 1 ( Fig. 3b ). The anomaly of FWHM (slope change 1,100–1,200 K) upon heating was well reproduced reversely (760–830 K) during cooling, which implies the reversible structural changes. The hysteresis-like feature of the FWHM is reminiscent of the hysteresis in viscosity and heat capacity peaks. It is plausible that the substantial structural changes in the liquid have occurred, because the suspension of a few percent solid crystalline particles itself would be not sufficient [27] to be responsible for the drastic viscosity change of approximately two orders of magnitude. For a single-component system, FWHM characterizes the degree of ordering of the system where larger width indicates a more disordered state. However, in the multicomponent Vit.1, the anomalies observed at 760–830 K and 1,100–1,200 K are probably not due to the behaviour of the width of a single peak but are more likely due to the shift of multiple underlying peaks, which is consistent with the behaviour of Q 1 and suggests that medium-range order atomic reconfiguration has occurred. Besides, from the G(r) data ( Supplementary Fig. S3 ), we noticed that the thermal behaviour for the higher-order coordination shell distances, r 2 , r 3 and r 4 , differ in an opposite way from the 1st shell distance r 1 which notably increases with decreasing temperature. The behaviour of r 1 suggests the increasing size of the short-range order clusters with decreasing temperature. A possible scenario is that when the size of the clusters approaches a critical value, this triggers the reconfiguration of the clusters packing on the medium-range order length scale, which might be related to the LLT. Liquid Vit.1 apparently fits into the strong class of Angell’s fragility pattern [21] and is comparable to the archetypal strong liquids, SiO 2 and BeF 2 , as well as water that are involved in a LLT [6] , [7] , [48] . Liquid SiO 2 is an extreme case of a strong liquid in the ‘strong/fragile’ pattern [21] . Saika-Voivod et al. [7] revealed a fragile-to-strong transition associated with a heat capacity anomaly above the melting temperature T m by studying static and dynamic properties of liquid silica using numerical simulations. Analogous to SiO 2 , molten BeF 2 studied by Hemmati et al. [8] using the ion dynamics simulations exhibits, also, a fragile-to-strong crossover as a result of a heat capacity maximum above T m . The experiments available for measuring the heat capacity maximum were carried out by Oguni and co-workers [17] , [49] using the supercooled water confined within silica gel nanopores to avoid crystallization. A pronounced heat capacity peak is observed at about 225 K above T g and below T m and is accompanied with a fragile-to-strong transition evidenced by a number of studies [16] , [20] . In another case of strong liquid As 2 Se 3 , a ‘semiconductor–metal’ transition was reported at high temperatures [50] , which are reminiscent of the LLT in SiO 2 and BeF 2 . The c p peak in Vit.1 with the strong-fragile crossover exhibits the similar behaviour to that of simulated SiO 2 and BeF 2 above T m and is comparable to water below T m . For comparison, c p versus T g -scaled temperature for Vit.1, SiO 2 (refs 51 , 52 ), BeF 2 (refs 8 , 53 ) and nanoconfined water [17] are plotted in Fig. 4 , also with the c p of a non-liquid superlattice system Fe 50 Co 50 (refs 13 , 55 ), which discloses a glass transition (kinetic freezing-in) during the lambda transition [13] . It is demonstrated [13] that the anomalous c p peak of these substances resembles a system with a lambda transition that is driven into off-critical behaviour, for example, by increasing the pressure (see inset in Fig. 4 ). This is reminiscent of the c p behaviour found in the simulations with the Jagla model including a LLCP that provides a mechanism for LLT [14] . It is hypothesized that LLTs are indeed underlying lambda transitions that separate a strong liquid below the transition temperature from a fragile liquid above it [13] . Consequently, strong liquids are expected to experience such a transition above T g , which can be observed when the observation window is appropriate and crystallization is avoided. This hypothesis is supported by the study of the present system where the kinetically strong system experiences a first-order transition corresponding to isobarically crossing a coexistence line with a possible underlying LLCP. In summary, our findings provide experimental support for the hypothesis [13] that the strong kinetics (low fragility) of a liquid arises from an underlying lambda LLT above T g . Thus, we expect to observe LLT also in other strong BMG-forming liquids [24] , [56] above their respective T g , if crystallization is avoided. Our study provides an important approach to experimental explorations of the LLT in metallic glass-forming systems and the LLT-correlated properties. Heat capacity measurements The amorphous Vit.1 samples were supplied by Liquidmetal Technologies. The sample rod was cut into disks with a mass ~60 mg to ensure good signals obtained from the calorimeter. The heat capacity was measured in reference to standard sapphire using graphite crucibles, in a high-purity argon atmosphere, with Netzsch STA 449/C/6/MFC/G Jupiter DSC-Cp mode. The c p peak was reproduced in tungsten crucibles to ensure it is not an effect of reaction with crucibles. The heat gain Δ H LL ≈1.0±0.1 kJ g-atom −1 is the mean value of the integrals of the c p peak areas of amorphous samples measured at different rates. Electrostatic levitation The electrostatic levitation experiments utilize electrostatic force generated by high-voltage amplifiers to levitate samples against gravity under high-vacuum (in the range of ~10 −7 mbar) conditions [57] (ref 57). Heating of the sample is achieved by infrared lasers. The sample is cooled continuously by switching off the laser power. Temperature of the sample was measured using pyrometry. The typical sample size is in the range of ~10–100 mg for both density and in situ XRD experiments. In situ X-ray-scattering experiment The in situ X-ray-scattering experiment was carried out on the beamline BW5 at HASYLAB/DESY in Hamburg. The beam size was 0.5*0.5 mm 2 and the X-ray wavelength was 0.124 Å (100 keV). Diffraction was performed in transmission mode using a Perkin Elmer 1621 AN/CN Digital X-ray detector with 2048*2048 pixels, pixel size 200*200 μm 2 . For isothermal measurements, samples were heated to the desired temperature, and 10 two-dimensional diffraction patterns were taken with an exposure time of 1 s for one frame. For continuous heating and cooling experiment, we acquired data with temporal resolution of 1 s. The cooling/heating and the recording of diffraction patterns were started simultaneously with 1 s exposure time as well. The correlation between temperature and the diffraction patterns was verified additionally at the temperature where crystallization of the sample sets. The pyrometer temperature was corrected according to the calorimetric onset of melting temperature of the sample assuming a constant emissivity. The uncertainty in the sample temperature determination resulted from the temperature versus diffraction pattern correlation and the pyrometer correction is estimated to be ±10 K. The total structure factors S(Q) were obtained from the integrated intensities I(Q) after the correction of Laue diffuse scattering and normalization to the atomic X-ray form factor, where I(Q) were obtained from the two-dimensional XRD patterns after background subtraction and corrected for sample absorption, fluorescence and inelastic (Compton) contribution using the data analysis software Fit2D [58] and PDFgetX2 (ref. 59 ). Detailed correction steps can be found in Egami and Billinge [46] . The positions of total structure factor maximum and reduced total pair distribution function maximum are extracted by a cubic spline interpolation method, which we find the most reliable way for the present liquid system. The FWHMs are obtained by fitting the data with Gaussian function. Volume measurements Volume measurements were performed on the levitated sample in the ESL by recording back-lighted sample images during continuous cooling and heating of the sample using a high-speed camera with 200 frames per second. The volume of the sample was then calculated according to the area of its shadow assuming rotational symmetry and calibrated with standard spheres with known volumes. For each data point, an average over 20 images was taken. Sample temperature is assumed to be constant during this time (0.1 s). Applying Yavari’s hypothesis According to the hypothesis of Yavari et al. [33] , Q 1 is associated with the change of the mean atomic volume V , and the temperature dependence of Q 1 ( T ) could be described by: where is the volume thermal expansion coefficient as determined by XRD. The best fit of the data ( Fig. 3b ) in the temperature range 850–1,300 K is given by α XRD ≈9.20 × 10 −5 K −1 . In light of their result for the amorphous state, the thermal expansion coefficient obtained from the XRD is the same as that measured in a dilatometer. However, for the liquid state of Vit.1, the thermal expansion coefficient from the XRD is different from that determined from a macroscopic volume measurement. How to cite this article: Wei, S. et al. Liquid–liquid transition in a strong bulk metallic glass-forming liquid. Nat. Commun. 4:2083 doi: 10.1038/ncomms3083 (2013).